Clustering in community structure across replicate ecosystems following a long-term bacterial evolution experiment Experiments to date probing adaptive evolution have predominantly focused on studying a single species or a pair of species in isolation. In nature, on the other hand, species evolve within complex communities, interacting and competing with many other species. It is unclear how reproducible or predictable adaptive evolution is within the context of a multispecies ecosystem. To explore this problem, we let 96 replicates of a multispecies laboratory bacterial ecosystem evolve in parallel for hundreds of generations. Here we find that relative abundances of individual species vary greatly across the evolved ecosystems and that the final profile of species frequencies within replicates clusters into several distinct types, as opposed to being randomly dispersed across the frequency space or converging fully. Our results suggest that community structure evolution has a tendency to follow one of only a few distinct paths. Although research is abound focusing on the adaptive evolution of a single species or a pair of interacting species, the problem of how evolutionary processes shape a complex natural ecosystem has received less attention [1] . Given the initial biotic and abiotic components of an ecosystem, it is not obvious whether we can ever predict the future community structure and species distribution for that ecosystem [2] . Resolving this challenging problem about community evolution is not only important from an intellectual standpoint, but also has implications for our ability to forecast the evolutionary responses of ecosystems to recent anthropogenic pressures [3] . Traditionally, research has pointed to character displacement, whereby co-occurring similar species diverge in their adaptations, and co-evolution as mechanisms to explain and predict adaptation in simple communities [2] . However, recent theory and experiments suggest that such predictions from niche occupancy patterns or pairwise species interactions often fail to predict adaptive evolution in more complex ecosystems composed of more than two species [4] , [5] . For instance, a recent experimental study with microbes found that community complexity can greatly alter adaptive evolution in a way that is not obvious from single-species evolution [6] . Diffuse co-evolution studies have also found evidence that co-evolution of a focal pair of interacting species can be influenced by the presence of other species [5] , [7] . All of these and similar studies mainly strive to elucidate deterministic mechanisms for multispecies adaptive evolution. However, we may also ask, to what degree is there randomness in the path that a multispecies ecosystem follows through adaptive evolution? If we could replay the evolution in a closed community many times starting from the same initial state, would we always end up in the same final state with the same abundances and kinds of species? Or would we get a different result each time? Recent theoretical and empirical studies using a single species suggest that adaptive diversification can be a surprisingly deterministic evolutionary process [8] , [9] . However, how this relates to multispecies adaptive evolution is less clear [2] . To address this problem, here we present experiments probing the adaptive evolution of a multispecies model community. We found evidence that the adaptive evolution of this experimental community is not deterministic, yet at the same time is not completely random. Our model community consisted of six soil bacteria species spanning three different genera: Enterobacter aerogenes (EA), Serratia marcescens (SM), Pseudomonas fluorescens (PF), Pseudomonas aurantiaca (PA), Pseudomonas veronii (PV) and Pseudomonas putida (PP). We let this community evolve in a complex environment containing dozens of carbon sources that can be found in soil (see Methods) [10] . We chose the species on the criteria that they could grow together in our media without aggressively antagonizing each other via either predation or expression of antimicrobial compounds. The carbon utilization profiles for these species were not completely overlapping, but also not fully orthogonal ( Supplementary Fig. 1 ). Compared with natural ecosystems with complex trophic levels and numerous types of species interactions, our model ecosystem is a simple one, where we expect most of the interactions between species to be driven by competition for resources [11] . To quantify the effect of evolution, we decided to look at community structure as a ‘trait’ for the ecosystem. We measured how this trait evolved across many replicates of the same initial ecosystem. We expected there to be three classes of possible outcomes: [1] replicate communities starting from the same initial state of community structure could simply diffuse in the frequency space and diverge randomly [2] , the replicates could altogether evolve to a new distinct state or [3] certain fractions of the replicates could evolve to different states leading the clusters across replicates ( Fig. 1 ). In our experiments, we observed the latter result. 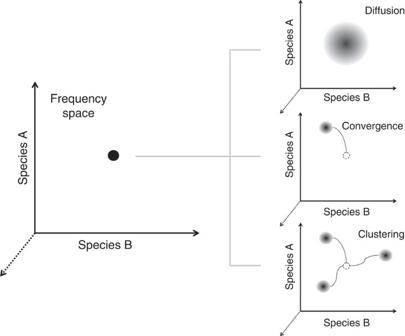Figure 1: Community structure as an evolving trait. If we start out with many replicates of the same ecosystem (which have the same initial community structure state, that is, the black cluster in the graph on the left), how would those replicates move in the frequency space over evolution? Possible scenarios are: (1) the replicates could simply diffuse in this space leading to a random divergence and increase in variation across replicates. (2) All the replicates could evolve in the same direction ultimately converging on a common final state, which is different from the initial state or (3) certain fractions of the replicates could evolve coherently in different directions leading to clustered final states after evolution. Experimentally we observed the latter case. Figure 1: Community structure as an evolving trait. If we start out with many replicates of the same ecosystem (which have the same initial community structure state, that is, the black cluster in the graph on the left), how would those replicates move in the frequency space over evolution? Possible scenarios are: (1) the replicates could simply diffuse in this space leading to a random divergence and increase in variation across replicates. (2) All the replicates could evolve in the same direction ultimately converging on a common final state, which is different from the initial state or (3) certain fractions of the replicates could evolve coherently in different directions leading to clustered final states after evolution. Experimentally we observed the latter case. Full size image Long-term evolution experiment We began by characterizing the relative abundance of the six bacterial species when mixed together. We prepared 96 identical ecosystems containing all six species, which we will refer to as the ancestral communities. We then allowed these ecosystems to reach (short-term) equilibrium by propagating through four growth dilution cycles. Each cycle of growth was approximately 10.5 cellular divisions per cycle. We were able to quantify the final species abundance by plating the communities on solid agar media and counting the colony numbers for each species, as each species had a unique colony colour/morphology ( Fig. 2a ). We found that Pseudomonas putida (PP) quickly fell to less than 1% abundance, whereas the other species were all between 15–35% in frequency. This coexistence of five of the six bacterial strains was observed in all 96 of our replicate ecosystems, suggesting that the short-term equilibrium of this ecosystem is reproducible and robust to experimental procedures and errors in measurement. 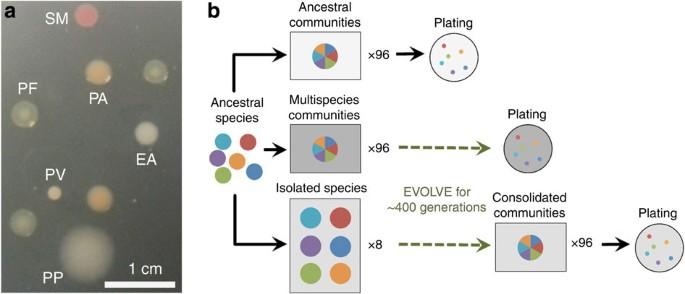Figure 2: Species appearance on an agar plate and evolution experiment design. (a) A photograph of colonies of all six species spread plated on an agar plate. Note the distinct colours and sizes of colonies, which enabled us to distinguish between the species (EA:Enterobacter aerogenes, SM:Serratia marcescens, PF:Pseudomonas fluorescens, PA:Pseudomonas aurantiaca, PV:Pseudomonas veroniiand PP:Pseudomonas putida). (b) This schematic shows the different treatments of the evolution experiment and how they were prepared. Ancestral species were mixed to create ancestral communities. For the multispecies treatment, again ancestral species were mixed together to establish 96 identical multispecies communities, but this time they were propagated as part of the long-term evolution experiment. For the isolated treatment, ancestral species were inoculated separately to create ‘isolated’ lines with eight replicates for each species and propagated along with the multispecies treatment. These long-term evolution treatments were propagated for ~400 generations corresponding to 42 cycles of transfers into fresh media every 48 h. In the end, multispecies communities were plated to measure relative abundance of species in each of the 96 replicates. Isolated lines were consolidated to make 96 multispecies communities. These consolidated communities from isolated lines were propagated for a short time and then plated for measurements. Figure 2: Species appearance on an agar plate and evolution experiment design. ( a ) A photograph of colonies of all six species spread plated on an agar plate. Note the distinct colours and sizes of colonies, which enabled us to distinguish between the species (EA: Enterobacter aerogenes , SM: Serratia marcescens , PF: Pseudomonas fluorescens , PA: Pseudomonas aurantiaca , PV: Pseudomonas veronii and PP: Pseudomonas putida ). ( b ) This schematic shows the different treatments of the evolution experiment and how they were prepared. Ancestral species were mixed to create ancestral communities. For the multispecies treatment, again ancestral species were mixed together to establish 96 identical multispecies communities, but this time they were propagated as part of the long-term evolution experiment. For the isolated treatment, ancestral species were inoculated separately to create ‘isolated’ lines with eight replicates for each species and propagated along with the multispecies treatment. These long-term evolution treatments were propagated for ~400 generations corresponding to 42 cycles of transfers into fresh media every 48 h. In the end, multispecies communities were plated to measure relative abundance of species in each of the 96 replicates. Isolated lines were consolidated to make 96 multispecies communities. These consolidated communities from isolated lines were propagated for a short time and then plated for measurements. Full size image Next, we performed a long-term evolution experiment consisting of 96 identical replicates of the six species community and let these evolve in parallel for ~400 generations, which we call the ‘multispecies evolution’ treatment ( Fig. 2b ). At the end of the experiment, we measured the final community structures (that is, the relative abundance of each species) in all communities. We found that all species except PP were very robustly coexisting in all of the replicate ecosystems. Surprisingly, in 9 out of the 96 ecosystems Pseudomonas putida (PP) not only survived the multispecies evolution process, but came to dominate the resulting communities ( Fig. 3c , mean frequency of ~25%). This stark bimodality in survival probability observed with PP may be due to a rare mutational event that occurred before PP went extinct. 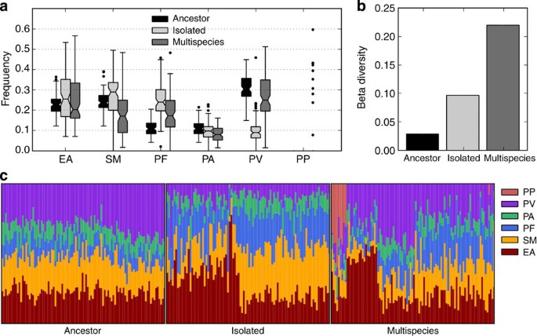Figure 3: Community structure outcomes look different across evolutionary treatments. (a) Box plots of relative abundance of each species for the replicates of different treatments. Note the 10 outliers in multispecies treatment for PP. (b) Beta diversity for different treatments, calculated using Jensen–Shannon divergence. Bars represent mean of 1,000 bootstrap runs with sample size 96 (with replacement), error bars too small to be visible (<1e−15). (c) Stacked area plots of raw relative abundance data for ancestral, isolated and multispecies treatments. Data are clustered and ordered using a hierarchical clustering algorithm to aid with visualization of distinct community structures. Horizontal axes represent observations (ancestor: 96 samples, cluster #k=2; isolated: 92 samples,k=2; multispecies: 96 samples,k=4). Figure 3: Community structure outcomes look different across evolutionary treatments. ( a ) Box plots of relative abundance of each species for the replicates of different treatments. Note the 10 outliers in multispecies treatment for PP. ( b ) Beta diversity for different treatments, calculated using Jensen–Shannon divergence. Bars represent mean of 1,000 bootstrap runs with sample size 96 (with replacement), error bars too small to be visible (<1e−15). ( c ) Stacked area plots of raw relative abundance data for ancestral, isolated and multispecies treatments. Data are clustered and ordered using a hierarchical clustering algorithm to aid with visualization of distinct community structures. Horizontal axes represent observations (ancestor: 96 samples, cluster # k =2; isolated: 92 samples, k =2; multispecies: 96 samples, k =4). Full size image In addition to evolution of the multispecies ecosystems, we in parallel performed isolated evolution of each of the individual species constituting this multispecies community (‘isolated evolution’). The isolated evolution treatment was designed to tease apart whether multispecies evolution was in any way different from the case where each species would evolve purely in response to the abiotic environment, irrespective of the presence of other species. After the long-term evolution experiment was over, we consolidated 96 multispecies communities using the species from the isolated treatment (see Methods). These new communities were grown for several cycles to reach equilibrium, after which we measured the final community structure by plating as we did for the multispecies treatment ( Fig. 2b ). Similar to the results with the ancestral communities, communities assembled using the isolated evolution lines yielded coexistence of species EA, SM, PF, PA and PV. Again, PP went extinct after a few cycles of growth in all communities (see Methods). The most striking difference in mean abundances was that the abundance of PV was significantly lower in the isolated treatment compared with both the multispecies and the ancestral treatment ( Fig. 3a ). The outcome of evolution in this new environment was therefore different depending on whether the species were co-evolving or evolving in isolation, in line with previous experimental results in a different microbial ecosystem [6] . A second notable feature of the relative abundance data was that PF was more abundant in the multispecies and isolated treatments than in the ancestral community. This might be due to some inherent advantage that this species possesses in terms of being able to adapt to this new environment. We also note that although we measure relative abundances (frequencies) of species in our experiments, these measurements can also be taken as a proxy for absolute abundance, since we did not observe any significant differences in final community productivity/optical density across treatments and replicates within each treatment ( Supplementary Fig. 2 ). The level of variation in relative species abundances across replicate communities also differed across the three treatments ( Fig. 3a ). Variation in species frequencies in the ancestral communities was much lower in comparison with the isolated and multispecies treatments, consistent with the expectation that adaptive evolution would increase community structure variation. Given that ancestral replicates were identical and had no time to evolve, variation in this treatment can be treated as a sum of measurement error and intrinsic fluctuations in the community structure. Therefore, by looking at the variation in the ancestral treatment, we can get a measure of this base error rate ( Fig. 3a , interquartile range: 6–8%). We also measured the beta diversity of each treatment as another measure of variation (Jenson–Shannon divergence, see Methods). We found that the multispecies treatment had a considerably higher beta diversity compared with both isolated and ancestral treatments ( Fig. 3b ). As discussed previously, PP went extinct in most of the multispecies community replicates (86/96; see Fig. 3c ), but when it survived, it came to dominate the community. This conclusion is also apparent looking at the raw frequency data plotted for each treatment ( Fig. 3c ). PP dominance is unique to the multispecies treatment. Clustering across replicates So far, we observed variation in community structure after adaptive evolution in multispecies and isolated treatments, and significantly more so in multispecies treatment. It is also important to determine whether there is anything deterministic about this variation. For instance, do the final community structures across replicates cluster into distinct types, where some fraction of the replicates converges onto the same community structure? If true, is there anything different between the treatments in terms of the cluster types and frequencies that we observe? To this end, we performed cluster analysis on our relative abundance data. We used consensus clustering, which provides quantitative and visual stability evidence for estimating the number of unsupervised classes in a data set [12] . Briefly, consensus clustering involves repeated subsampling of the data and then applying a clustering algorithm to each subsample (see Methods). In the case where there are very distinct clusters in the data, an observation in each subsample would always cluster with the same set of observations regardless of which portion of the whole data set we are using. Alternatively, if the clusters were not robust depending on the subsample, then the cluster assignment for each observation would vary. The ‘consensus’ score of two observations is essentially the frequency with which they cluster together. This score would be 1 if the two observations always clustered into same class in each subsample where both of them happened to be present. A clustering analysis of the relative species abundances from the multispecies evolution experiment argued that our 96 replicates could be divided into four distinct outcomes ( Fig. 4a ). Visual inspection of the heatmaps of consensus score matrices for different k ’s (number of clusters) suggested that the most clean matrix is for k =4, indicating that the optimal number of classes in this data set is 4 (for a more detailed analysis, see Supplementary Fig. 3 ). We also performed the same clustering analysis for the isolated evolution treatment, which indicated that the optimal clustering of this data is for k =2 ( Fig. 4b , Supplementary Fig. 4 ). The same analysis was performed for a randomly generated data set and the ancestral data set. The results from these analyses showed that multispecies treatment has a comparably higher clustering quality and larger number of distinct clusters ( Supplementary Figs 5 and 6 ). 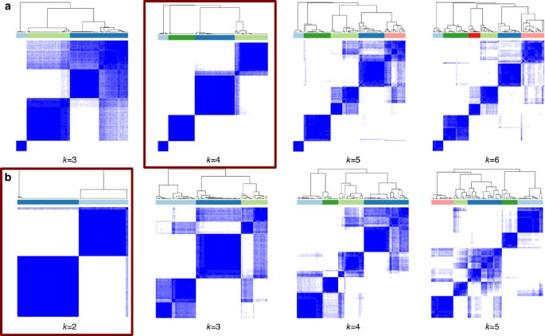Figure 4: Multispecies treatment results in higher number of distinct community structures as quantified by consensus clustering. (a) Consensus matrices for multispecies treatment. (b) Consensus matrices for isolated treatment.kvalues indicate number of clusters used ink-means algorithm. Rows and columns correspond to observations. Note that the cleanest matrix for multispecies treatment is atk=4, whereas for the isolated treatment it is atk=2 (indicated by big squares). Consensus values range between 0 and 1, coloured by white to dark blue. Scaling is the same across all plots. A consensus value of 1 for two items means these two items clustered together 100% of the time across all subsamples, whereas a value of 0 means that two items never clustered together. A dendrogram of consensus clustering results is plotted above the columns of the heatmaps, and the identified clusters are colour-coded. Figure 4: Multispecies treatment results in higher number of distinct community structures as quantified by consensus clustering. ( a ) Consensus matrices for multispecies treatment. ( b ) Consensus matrices for isolated treatment. k values indicate number of clusters used in k -means algorithm. Rows and columns correspond to observations. Note that the cleanest matrix for multispecies treatment is at k =4, whereas for the isolated treatment it is at k =2 (indicated by big squares). Consensus values range between 0 and 1, coloured by white to dark blue. Scaling is the same across all plots. A consensus value of 1 for two items means these two items clustered together 100% of the time across all subsamples, whereas a value of 0 means that two items never clustered together. A dendrogram of consensus clustering results is plotted above the columns of the heatmaps, and the identified clusters are colour-coded. Full size image We further evaluated the quality of clustering by looking at the mean cluster consensus for each treatment, where we took the mean of the average consensus scores for each cluster identified. We observed that mean cluster consensus values for both the ancestral and random data sets were lower compared with multispecies and isolated treatments, random data set being the least robust overall ( Supplementary Fig. 7A ). We also confirmed that our results were robust to the clustering method used, as similar cluster quality and number trends were observed with hierarchical clustering of the same data ( Supplementary Fig. 7B ). Taken together, these results suggest that adaptive evolution in our experimental system often resulted in one of several distinct community structure states in multispecies and isolated treatments, more so than would be expected by random variation. Moreover, multispecies treatment resulted in higher number of these states/clusters compared with the isolated treatment, suggesting that multispecies adaptive evolution might be less predictable compared with single-species evolution. This result is also consistent with the high beta diversity observed in the multispecies data set. Moreover, the larger number of clusters and higher beta diversity in the multispecies treatment is not due to any sampling effect that might have occurred with the way that the isolated treatment was designed (that is, six replicates for each isolated treatment), since subsampling from the multispecies treatment still yields a higher beta diversity than observed in the isolated treatment ( Supplementary Fig. 8 ). We also found that clusters in the multispecies and isolated treatments are distinct from the ancestral community structure ( Supplementary Fig. 9 ), with two clusters in multispecies treatment only partially overlapping with the ancestral treatment. Cluster behaviour is dominated by driver species Next, we wanted to understand the underlying mechanisms leading to this clustering effect. To address this question, we compared each cluster with the ancestral community structure ( Fig. 5a ). We quickly realized that each cluster was mostly defined by one single species doing significantly better compared with its counterpart in the ancestral community. The most extreme example of this occurred in cluster 1 where PP was present in very high frequency, whereas it was practically extinct in the ancestral community. Given this observation, we hypothesized that the behaviour of each cluster could be mainly driven by only one species (PP, EA, PV or PF) increasing in frequency, probably owing to a relatively rare mutation conferring a significant selective advantage. 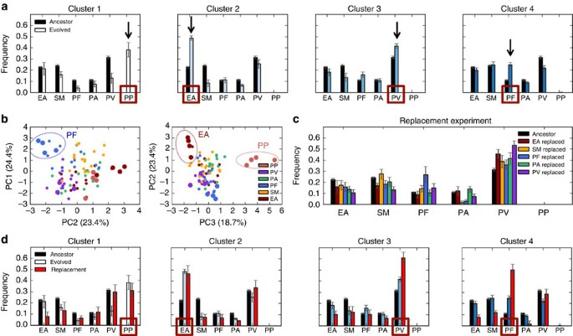Figure 5: Replacing ancestral species with evolved isolates in the ancestral community reproduces the clustering behavior. (a) Comparison of each cluster against ancestral community (n=9 for cluster 1,n=18 for cluster 2,n=22 for cluster 3,n=47 for cluster 4. Species that are significantly higher in frequency compared with their ancestral level are indicated with arrows. (b) Principal component analysis (PCA) plots for replacement experiment data. Each circle represents an ancestral community in which a species is replaced with an evolved isolate from the multispecies treatment. Circles are colour-coded based on the species that is replaced in the ancestral community. Big circles represent communities in which ancestral species are replaced with evolved isolates that were highlighted ina, driver isolates. (c) Mean relative abundance for the communities shown in PCA analysis inb, excluding driver isolates. (d) Comparison of each cluster against ancestral community and the communities created by replacement with the driver isolates froma(big circles inb). Replaced species are highlighted in squares on thexaxis labels, error bars are 95% confidence interval around mean. Figure 5: Replacing ancestral species with evolved isolates in the ancestral community reproduces the clustering behavior. ( a ) Comparison of each cluster against ancestral community ( n =9 for cluster 1, n =18 for cluster 2, n =22 for cluster 3, n =47 for cluster 4. Species that are significantly higher in frequency compared with their ancestral level are indicated with arrows. ( b ) Principal component analysis (PCA) plots for replacement experiment data. Each circle represents an ancestral community in which a species is replaced with an evolved isolate from the multispecies treatment. Circles are colour-coded based on the species that is replaced in the ancestral community. Big circles represent communities in which ancestral species are replaced with evolved isolates that were highlighted in a , driver isolates. ( c ) Mean relative abundance for the communities shown in PCA analysis in b , excluding driver isolates. ( d ) Comparison of each cluster against ancestral community and the communities created by replacement with the driver isolates from a (big circles in b ). Replaced species are highlighted in squares on the x axis labels, error bars are 95% confidence interval around mean. Full size image To test this hypothesis, we collected isolates for each species from each cluster in the multispecies treatment (four randomly chosen communities per cluster and 3–5 pooled colonies per species in each community, giving 4 clusters × 4 communities × 5 species=80 isolates plus 4 PP isolates from cluster 1, totalling 84 isolates). We then systematically created communities where each evolved isolate replaced its counterpart species in the ancestral community ( n =84). We then grew these communities to equilibrium and measured relative abundances. A principal component analysis (PCA) of the resulting species abundances was consistent with our hypothesis that the clusters were largely driven by adaptive evolution of the common species from each cluster. Given this hypothesis, we expected to see clusters in PCA plots due to the distinct behaviour of communities assembled with isolates we thought were driving the behaviour of each cluster (for example, PP from cluster 1, EA from cluster 2 and so on). Indeed, we found that communities assembled with PP isolates from cluster 1, EA isolates from cluster 2 or PF isolates from cluster 4 had distinct community structures and clustered separately in PCA plots (big circles in Fig. 5b ). However, we did not observe a separate cluster corresponding to communities prepared with PV isolates from cluster 3. When we compared all the communities excluding the ones assembled with our hypothesized ‘driver’ isolates (big circles in Fig. 5b ) against the ancestral community structure, we found that there was little difference ( Fig. 5c ). The only exceptions were that communities with PF or PV isolates did in general have higher PF or PV frequencies respectively, compared with the ancestral community. This observation suggests that in all the clusters, there might be across the board adaptation within the context of certain species. Finally, we compared the ancestral communities assembled with our hypothesized driver isolates (PP from cluster 1, EA from cluster 2, PV from cluster 3, PF from cluster 4) with the evolved clusters and the original ancestral community. We found that we could reproduce the qualitative behaviour of each cluster observed in multispecies treatment ( Fig. 5d ). In conclusion, these results suggest that the significant clustering we observed was the result of a single species gaining an advantage and increasing in frequency in each cluster. This strong effect seemed to produce divergent states in the community structure across replicates, because in each distinct outcome a different species was more abundant. Here we developed an experimental model ecosystem that exhibits robust coexistence of 5–6 soil bacteria species. This system allowed us to perform highly parallel long-term co-evolution experiments. In the end, we found that although there is variation in the final outcome of adaptive community evolution, the final community structure seems to end up in one of a few distinct states. Moreover, these final states depend on whether the evolution occurred in a multispecies community or as isolated single species, suggesting that multispecies ecosystem evolution is fundamentally different from species evolving by themselves. We found that the discrete states we observed after multispecies evolution are the result of a different species doing substantially better than others in each case. It would be interesting to probe even longer term co-evolution, as the ‘final’ ecological states that we have examined here are of course simply a snapshot in time of the co-evolutionary process. Moreover, it could be that the outcomes we observed are communities on various stages along a transition from an ancestral type, in which different numbers of mutations have already arisen and spread. We can ask whether the large changes in community structure that we observed are really due to evolution as opposed to being manifestations of different stable ecological states. First, if the latter were true, we would expect to observe such variation in ancestral communities or consolidated isolated lines. Instead, ancestral communities displayed no significant clustering or variation and the isolated treatment had only two clusters compared with the four observed in the multispecies treatment. These results are also in line with our repeated observations with ancestral lines where, independent of the initial inoculation frequencies of the species, the measured community structures were invariably the same after a few cycles of transfers. Moreover, replacement experiments showed that by using isolates from evolved communities, we could reproduce the community structures observed at the end of the evolution experiment, suggesting that the changes in community structure were driven by evolutionary responses rather than stochastic fluctuations. The predictability of adaptive evolution is a fundamental question that has puzzled evolutionary biologists since Darwin [13] . Studies investigating the determinism of adaptive evolution have historically focused on adaptive radiation of single species into new environments. For instance, more than a decade ago, researchers reported that replicated adaptive radiations of island lizards indicate that adaptive radiation follows deterministic paths resulting in convergent evolution [14] . Since then, subsequent studies using lizards or other animals have reinforced these results [15] , [16] , [17] , [18] . In addition to such animal studies, microcosm experiments have also pointed to similar conclusions. Evolution experiments using organisms like Escherichia coli or viral models found evidence of parallel evolution, whereby replicate populations evolved convergent characteristics when adapting to new environments [9] , [19] , [20] , [21] , [22] . Similarly, instances of parallel evolution have also been observed among higher organisms like plants and insects and also in nematode development [23] , [24] , [25] , [26] . These studies suggest that at least within the context of a single species, evolution can be surprisingly deterministic and convergent. In contrast to these previous studies, our experiments looked at adaptive evolution of a multispecies community rather than focusing on a single species. We found that this multispecies aspect can result in a less predictable outcome of adaptive evolution than single-species studies would suggest. Even without external perturbations or environmental fluctuations, we observed intrinsic randomness in evolution that comes with having a multispecies ecosystem. Nevertheless, we still found that the adaptive community evolution is not completely random and final community structures cluster into several distinct types. We speculate that the high variation in community structure observed in natural microbial ecosystems, such as human microbiota samples, might be partially due to evolutionary processes similar to what we have observed in our experiments [27] . However, more laboratory experiments and data from wild populations are needed to validate the generality of our results. Experiments using tractable multispecies ecosystems like ours can improve our understanding of the predictability of community structure evolution. Species and media The six soil bacteria species we used were Enterobacter aerogenes (ATCC#13048), Serratia marcescens (ATCC#13880), Pseudomonas fluorescens (ATCC#13525), Pseudomonas aurantiaca (ATCC#33663), Pseudomonas veronii (ATCC#700474) and Pseudomonas putida (ATCC#12633), and they all were obtained from ATCC. The growth media was prepared using commercially available BIOLOG EcoPlates. These microplates contain 31 different carbon sources useful for soil community analysis. In addition to these carbon sources, in each well there is a tetrazolium dye (5 cyano-2,3 ditolyl tetrazolium chloride), which is reduced to a violet-fluorescent formazan molecule, when the carbon source is oxidized by the cells. The colour development was measured by light absorption at 590 nm, which quantified the productivity of cultures. At the same time, the optical density of the cultures was measured at 750 nm, where the tetrazolium dye is not absorbent. Our base media was M9 minimal media, which contained 1X M9 salts (Sigma Aldrich), 2 mM MgSO 4 , 0.1 mM CaCl 2 , 1X trace metals (Teknova). We filled the EcoPlate by adding 140 μl of this base media into each well and let the lyophilized carbon sources dissolve for 30 min. Then, we mixed all the contents of the wells (except the blanks) to get a complex medium containing all of the 31 carbon sources. For initial inoculation and growth of the species before experiments, we used nutrient broth (0.3% yeast extract, 0.5% peptone). We used nutrient agar plates (nutrient broth+1.5% agar) to count colonies and measure the relative abundances of species. All experiments were done at 24 °C. Evolution experiment From frozen stocks of ancestral lines, we directly inoculated each species separately into nutrient broth and let them grow for 48 h in loose-cap culture tubes without shaking. Next, we inoculated the grown cultures into our base media and again let the species grow separately for two cycles of transfers (48 h each). We diluted these by 1/100 into M9 minimal media (w/o carbon sources) then added 10 μl of this mixture onto 140 μl of our base media corresponding to 1/1,500 dilution in total. These cultures were inoculated into flat-bottom 96-well plates, every well of the microplate contained 150 μl of media plus cells. For each transfer, we diluted cultures by 1/1,500 into freshly prepared media. After this initial period of growth, we made frozen stocks of these cultures, and at the same time we initiated the two treatments of the long-term evolution experiment [1] : for the multispecies treatment, we diluted each of the individual species by 1/100 and then mixed them by equal volume. After this, we diluted that mixture by 1/15 into freshly prepared base media and then used this final mixture to inoculate the wells. We had 96 replicates for this treatment, and these replicates were spread over two 96-well plates using a checkerboard pattern to mitigate risk of cross-contamination [2] . For the isolated treatment, we diluted those same cultures for the individual species by 1/1,500 and had eight replicates for each species adding up to 48 cultures in total for six species. These were also spread over a 96-well plate in a checkerboard pattern. Throughout the course of the evolution experiment, every 48 h, cultures in both treatments were diluted by 1/1,500 into media that were freshly prepared just before the experiment. The cultures were incubated without orbital shaking. Measurements after the evolution experiment After 42 cycles of transfers, we measured the relative abundances in the multispecies treatment by plating on nutrient agar plates. For each replicate, we diluted the final cultures by 1/10 6 in phosphate-buffered saline, and plated 75 μl of this solution onto an agar plate. We plated each replicate twice, as during preliminary experiments, we found that there was large variation in the total number of colonies that showed up on plates. After 48 h, we counted all the colonies on two plates together to measure the relative species abundances. For each replicate at least ~90 colonies were counted. We confirmed evolved species identities for at least 20 communities by checking carbon utilization profile of each species isolate on Biolog Ecoplates. We also plated all 48 cultures in the isolated evolution treatment to check for possible contamination. We found that two replicates of one of the species (PA) had no colonies on agar plates possibly due to external contamination. We discarded these replicates and used the remaining ones. We also made frozen stocks for all of these final cultures. To prepare the consolidated communities for the isolated treatment, we randomly chose six of the eight replicates for each species. We chose six to balance out the fact that we had only six viable replicates for one of the species (PA). Next, after inoculation into base media from frozen cultures and growth for two cycles, we randomly chose a replicate from the six replicates for each species and mixed them equally by volume, then repeated this process for 96 times to get 96 randomly consolidated communities using the species from the isolated evolution. We diluted these communities by 1/1,500 into fresh media and let them grow for four cycles of transfers, after which we plated them and measured the relative species abundances as we have done for the multispecies treatment. We found that four of these cultures had no growth in the end, so we used the remaining 92 for our measurements. We got visible PP survival only in three of the communities but in very low abundance (~1%, one colony in ~100). To see if this was due to the initial mixing ratios we had used, we repeated consolidation again using the same procedure of random mixing but this time instead of using 1/6 of volume for PP, we used a proportionately excess amount of 1/4 in volume while the other species equally occupied the other 3/4. After four cycles of growth, PP was visible only in six communities but was still less than 3% in frequency. We decided to use the initial data set where we had initially mixed all the species by equal volume, as there was no appreciable effect of increasing the initial frequency of PP. For preparing the ancestral communities, we revived the frozen stocks of ancestral species that were stored during the initiation of the evolution experiment and let them grow in base media for two cycles then mixed them by equal volume, and created 96 replicate communities. After four cycles of transfers of these communities, we plated them and measured relative species abundances. PP colonies were found in four communities, but we could count only one or two colonies per plating in all of these cases. We did not observe any significant difference in community structure with or without PP, either for ancestral communities or for the communities created using isolated lines. Therefore, for our analyses with the ancestral and isolated treatments, we assume that PP is essentially extinct and exclude PP data, also taking into account that these low-frequency measurements could be false positives. We also note that our measurement resolution was not sufficient enough to measure frequencies lower than ~1%, but PP could still be surviving in lower frequencies in these experiments albeit not detectable by our measurements. In Fig. 3 , Jensen–Shannon divergence is where H is Shannon entropy and C i is the community structure of i th replicate. Cluster analysis For consensus clustering, we used k -means clustering algorithm with Pearson distance. In total, 80% of the data were subsampled without replacement for a total of 100 iterations. This process was repeated for each k (number of clusters) and the results from these were used to create consensus matrices and calculate mean consensus values for each class and each observation in the data set. Items or clusters were not weighted in the subsamples. We generated a random data set by creating 96 artificial observations, where each observation contained five frequency variables, as in our actual relative abundance data sets. These frequency values were assigned by drawing from a uniform distribution and then normalizing across each observation. Having six frequency variables instead of five did not change the results. Hierarchical clustering was performed using Euclidean distance and ‘ward’ linkage. Calinski–Harabasz index is a measure of the ratio of inter-cluster variation to within cluster variation, hence the larger this number is the better the cluster separation and cluster compactness. These analyses were performed using R statistical language and open source packages [12] , [28] . Replacement experiments At the end of the evolution experiment, we froze all the communities as mentioned previously. To perform the replacement experiments, for each identified cluster in the multispecies treatment, we inoculated four randomly selected communities into fresh media from the frozen stocks (4 × 4=16 communities). We propagated these cultures for four cycles of transfers using the same scheme we had in the long-term evolution experiment. Then, we plated these 16 communities and picked 3–5 colonies per species from each plate. We pooled the picked colonies for a given species from a plated community and then inoculated those into fresh media (five species per plate from clusters 2, 3, 4; and six species per plate from cluster 1, that is, 3 clusters × 4 communities × 5 species=60 isolates in total from clusters 2, 3, 4; plus 1 cluster × 4 communities × 6 species=24 isolates from cluster 4). We let these isolates grow for two cycles. For the replacement experiment, we mixed each isolate with its complementary ancestral species (which were also grown for two cycles in parallel with isolates). For instance, for an EA isolate, we mixed it with ancestral species SM, PF, PA, PV. We again let these newly prepared communities grow for four cycles of transfers before we plated them to measure relative abundances. How to cite this article: Celiker, H. and Gore, J. Clustering in community structure across replicate ecosystems following a long-term bacterial evolution experiment. Nat. Commun. 5:4643 doi: 10.1038/ncomms5643 (2014).